Measurement of the inelastic proton–proton cross-section at √s=7 TeV with the ATLAS detector The dependence of the rate of proton–proton interactions on the centre-of-mass collision energy, √ s , is of fundamental importance for both hadron collider physics and particle astrophysics. The dependence cannot yet be calculated from first principles; therefore, experimental measurements are needed. Here we present the first measurement of the inelastic proton–proton interaction cross-section at a centre-of-mass energy, √ s , of 7 TeV using the ATLAS detector at the Large Hadron Collider. Events are selected by requiring hits on scintillation counters mounted in the forward region of the detector. An inelastic cross-section of 60.3±2.1 mb is measured for ξ>5×10 −6 , where ξ is calculated from the invariant mass, M X , of hadrons selected using the largest rapidity gap in the event. For diffractive events, this corresponds to requiring at least one of the dissociation masses to be larger than 15.7 GeV. Since the earliest days of particle physics, measurements of the total pp and pp̄ cross-sections and their theoretical understanding have been topics of much interest [1] . The cross-sections cannot yet be calculated by quantum chromodynamics, and many approaches have been used to describe the existing measurements. General arguments based on unitarity and analyticity imply a bound (the Froissart bound [2] , [3] ) on the high-energy behaviour of total hadronic cross-sections. This bound is independent of the details of the strong interaction dynamics and states that the total cross-section cannot rise faster than ln 2 ( s ), where √ s is the centre-of-mass energy. Recently, it has been extended to the inelastic cross-section [4] . Existing experimental data [1] show a rise in the hadronic cross-sections with s , but it is unclear whether the asymptotic behaviour has already been reached. In this letter, a direct measurement of the inelastic pp cross-section at the highest energy collider to date is presented. Measurements of the inelastic p -air cross-section in the multi-TeV regime are available from cosmic-ray shower detection experiments [5] , [6] , [7] , [8] , and have been used to infer the pp cross-section albeit with significant uncertainties. The measurement presented here is of direct relevance for the modelling of high energy cosmic ray showers. The most common models that describe the data up to TeV predict a rise of the total cross-section with a simple power law ( s α (0)–1 where α (0) denotes the Pomeron-trajectory intercept) [9] , [10] , [11] or with a power law depending on ln( s ) (refs 12 , 13 , 14 , 15 , 16 ). Others employ quantum chromodynamics for aspects of the calculation [17] , [18] , [19] , [20] . However, although the phenomenological description of the existing data is largely adequate, there are significant uncertainties on the extrapolation to higher energies, partly due to a long-standing 2.7σ discrepancy between the two highest energy collider measurements of the total pp̄ cross-section by CDF [21] and by E811 (ref. 22 ). The inelastic pp cross-section at TeV is measured with data taken by the ATLAS experiment [23] at the Large Hadron Collider (LHC) [24] . The data considered were collected during a single 8-hour fill beginning 31 March 2010, corresponding to an integrated luminosity of 20.3±0.7 μb −1 and a peak instantaneous luminosity of 1.2×10 27 cm −2 s −1 . The mean number of interactions per crossing in this fill is ∼ 0.01. The analysis uses highly efficient scintillation counters, the minimum bias trigger scintillator (MBTS) detectors, to detect inelastic collisions. They are insensitive to diffractive dissociation processes in which the dissociation systems have small invariant masses, M X . Their acceptance corresponds approximately to ξ= M X 2 / s >5×10 −6 , equivalent to M X >15.7 GeV for TeV. The cross-section measurement presented here is restricted to this kinematic range. However, to compare the data with previous measurements, an extrapolation of the cross-section is performed to the full ξ range, ξ > m p 2 / s where m p is the proton mass. Acceptance determination Monte Carlo (MC) simulations are used to determine the acceptance of the event selection and to assess systematic uncertainties. The detector response to the generated events is simulated using the ATLAS simulation [25] based on Geant4 (ref. 26 ), and both the simulated and data events are reconstructed and analysed with the same software. The Pythia6 (ref. 27 ), Pythia8 (ref. 28 ) and Phojet [29] , [30] generators are used to predict properties of inelastic collisions. These generators distinguish between different processes that contribute to inelastic pp interactions: single dissociative (SD) processes, pp→pX , in which one proton dissociates; double dissociative (DD) processes, pp→XY , in which both protons dissociate with no net colour flow between the systems X and Y ; and non-diffractive (ND) processes in which colour flow is present between the two initial-state protons. The model by Schuler and Sjöstrand [31] , used by Pythia6 and Pythia8, predicts cross-sections of 48.5, 13.7 and 9.3 mb for the ND, SD and DD processes, respectively. Whereas the cross-sections used by Pythia6 and Pythia8 are identical, they differ in the modelling of the hadronic final state. Phojet predicts the corresponding cross-sections as 61.6 mb (ND), 10.7 mb (SD) and 3.9 mb (DD). Because of differences in implementation of the interface between large ξ diffractive (SD and DD) processes and ND processes in Pythia and Phojet, the fractional contribution of these processes is a model-dependent quantity. Phojet also includes a 1.1 mb contribution from central diffraction (CD), pp→ppX , a process not implemented in Pythia, wherein neither proton dissociates, but the Pomeron–trajectory exchange results in energy loss for the protons and the production of a central system of particles. The MC generators define the inelastic cross-section as the sum of these contributions, and thus Schuler and Sjöstrand (Phojet) predicts an inelastic cross-section of 71.5 mb (77.3 mb). Other recent predictions for this cross-section at TeV are 69 mb (ref. 15 ), 65–67 mb (ref. 17 and personal communication with the author), 68 mb (refs 18 , 19 ) and 60–75 mb (ref. 20 ). Although the cross-section measured here is quoted for a restricted ξ -range, ξ is not directly measured. However, the η coverage of the MBTS implies a lower bound on the range of ξ -values for events that the detectors can observe. To study the acceptance as a function of ξ , MC generators are used. The variable ξ is defined at the particle level by dividing the final state particles from the MC generators into two systems, X and Y . The mean η of the two particles separated by the largest pseudorapidity gap in the event is used to assign all particles with greater pseudorapidity to one system and all particles with smaller pseudorapidity to the other [32] . The mass, M X,Y , of each system is calculated, and the higher mass system is defined as X while the lower mass system is defined as Y . In the case of SD, Y is the non-dissociated proton. The variable ξ is then given by ξ = M X 2 / s and it is bounded by the elastic limit, satisfying ξ> m p 2 / s . As expected from kinematic considerations, a strong correlation is observed, independently of the MC model used to determine ξ , between ξ and the pseudorapidity of the hadron from X that is farthest from the initial-state proton pseudorapidity. Therefore, the upper limit of the MBTS detector acceptance of | η |<3.84 (see Methods ) can be translated into a limit on the ξ of observed events. Thus the measurement is restricted in its ξ -range; there is no requirement on M Y . Several models are used for the dependence of the diffractive cross-sections on ξ . The Schuler and Sjöstrand model has a relatively flat dependence on ξ , whereas the Phojet model predicts a slight decrease with decreasing ξ . Pythia8 has several extra predictions for the ξ -dependence of the diffractive cross-sections that are considered. In the low ξ regime, Bruni and Ingelman [33] predict a flat ξ -dependence whereas Donnachie and Landshoff (DL) [34] and Berger et al . [35] predict where ɛ = α (0)−1. Values of ɛ between 0.06 and 0.10, and of α ′ between 0.10 and 0.40 GeV −2 are considered for the DL model. α ′ is the slope of the Pomeron trajectory that is assumed to be linear such that α ( t )= α (0)+ α ′ t . The DL model with ɛ =0.085 and α ′=0.25 GeV −2 with Pythia8 fragmentation is the default model in this analysis, and the other models are used to assess uncertainties in the modelling of diffractive events. Cross-section calculation elements Experimentally the cross-section is calculated using where N is the number of selected events, N BG is the number of background events, f ξ < 5 × 10 - 6 is the fraction of events that pass the event selection but have ξ<5×10 −6 , is the integrated luminosity, and ɛ trig and ɛ sel are the trigger and offline event selection efficiencies in the selected ξ -range. For ξ=5×10 −6 , ɛ sel is 50%, rising to nearly 100% for ξ >10 −5 . The dependence of the efficiency on ξ is similar for the SD and DD processes and for different MC generators. The measurement is quoted for ξ> 5×10 −6 that gives the smallest correction factor, and thus yields the smallest systematic uncertainty on the measurement due to the underlying ξ -distribution. In this measurement, N BG and ɛ trig are determined directly from the data. The MBTS individual counter efficiencies in the MC simulation are tuned to match the observed efficiencies in data. Then ɛ sel and f ξ < 5 × 10 - 6 are taken from the tuned MC simulation. To reduce the uncertainties in the factors taken from MC simulation, the relative diffractive dissociation cross-section, for each generator is constrained. Each of these steps is described in detail below. The MBTS functions as a trigger by determining the number of scintillation counters with a signal passing a leading-edge discriminator; in this analysis, at least one trigger signal must be present. In the offline reconstruction, the MBTS signals are fit to obtain the total charge and timing of the signal. The offline event selection requires at least two counters with a charge larger than 0.15 pC. This threshold is set to be well above the noise level, which is well described by a Gaussian centred at zero of width 0.02 pC. This inclusive sample contains 1,220,743 data events. To constrain the diffractive components, a subset of events that have at least two hits on one side of the MBTS detector and no hits on the opposing side (in z ) are selected. In the data, 122,490 of these single-sided events are observed. Backgrounds Backgrounds arise from beam-related interactions, such as collisions of the beam with gas particles in the beam-pipe or with material upstream from the detector, and slowly-decaying, collision-induced radiation termed 'afterglow' [36] . Additionally, instrumental noise and cosmic rays provide backgrounds that were studied and found to be negligible for this analysis. The beam-related backgrounds are determined using the number of selected events collected in this fill with the non-colliding bunches, that is, when only one proton bunch was passing through ATLAS [37] . They are normalized by the ratio of the number of protons in the colliding to the non-colliding bunches. The single-sided selection contains 422±28 background events and the inclusive sample contains N BG =1,574±54 background events, corresponding to 0.3% and 0.1% of the total samples, respectively. In addition, there is an in-time afterglow component owing to the scattering of secondary low-energy particles produced in the same collision event that can give extra hits, causing low-activity events to migrate into the selected event sample. This contribution is evaluated to be at most 0.4% for the inclusive, and 3.6% for the single-sided samples, by examining the asymmetry of the absolute timing measurement of the MBTS counters. We conservatively assume a 100% uncertainty on both background sources that covers any residual impact of the afterglow on the background subtraction, any uncertainty in the beam current measurements and the uncertainty due to in-time afterglow. The resulting overall uncertainty on the number of background events N BG is given by the quadratic sum of the two components and is 0.4%. Detector efficiency and modelling The trigger efficiency of the MBTS detector, with respect to the offline requirement, ɛ trig , is measured to be (statistical errors) using events triggered randomly on colliding beams. The systematic uncertainty on ɛ trig is determined using a second, independent trigger as reference. The difference between the two efficiency determinations leads to a 0.1% uncertainty on the cross-section measurement. The data and MC simulation agreement in the MBTS counter response is checked using other detector subsystems with overlapping η ranges: charged particles reconstructed by the tracking detector (2.09<| η |<2.5), and calorimeter showers in the inner wheel of the electromagnetic calorimeter (2.5<| η |<3.2) and in the forward calorimeter (3.1<| η |<3.84). The efficiency with respect to a track (calorimeter energy deposit) to have a signal above the 0.15 pC threshold in the outer (inner) counters is on average 98.5% (97.5%) for the data and a constant 99.4% (98.7%) in the MC simulation. The individual counter efficiencies deviate by up to 2.0% (2.5%) from the average in the data. The MC simulation is corrected to match the data efficiency, and the maximum variations in the counter responses are considered as a systematic uncertainty. This results in a 0.1% uncertainty on the cross-section measurement. The offline selection efficiency, ɛ sel , depends on the amount of material traversed by particles before hitting the MBTS detector. The rate of photons (primarily from π 0 decays) converting to electrons that are subsequently detected by the MBTS increases with extra material, resulting in an increase of ɛ sel . Second order effects arise from charged particles scattering out of the MBTS acceptance region (decreasing ɛ sel ), or charged particles scattering into the acceptance region (increasing f ξ < 5 × 10 - 6 ). Within the tracking volume (| η |<2.5), the material distribution has been studied using conversion electrons and decays, and is known to better than ±5% in the central region of the detector and to ±30% for 2.2<| η |<2.5 (ref. 38 ). In the region | η |>2.5, the material is dominated by the cooling and electrical services to the silicon pixel detector, and an uncertainty of ±40% is assumed. This is validated in-situ using the fraction of events wherein we observe significant energy in the forward calorimeters but no signal (above noise) in the MBTS detector. The resulting systematic uncertainty on the cross-section is 0.2%. Misalignments of the MBTS detector with respect to the nominal centre of the detector could change the event selection efficiency for a particular value of ξ . Misalignments of up to 10 mm were considered and found to have a negligible impact. A misalignment of 10 mm is conservative compared with the survey precision and any known misalignments within the ATLAS experiment [23] . Fractional diffractive event contribution The fractional contribution of diffractive events, f D , is constrained by the ratio of single-sided to inclusive events, R ss . The MC generators predict that less than 1% of the ND process pass the single-sided event selection, whereas 27–41% of the SD and DD processes pass the single-sided selection. For all models, the inclusive sample is dominated by ND events; therefore, the ratio of single-sided to inclusive events is sensitive to the relative fraction of diffractive events. The measured R ss in the data is where the systematic error includes the uncertainties on the backgrounds, the MBTS response and the material. 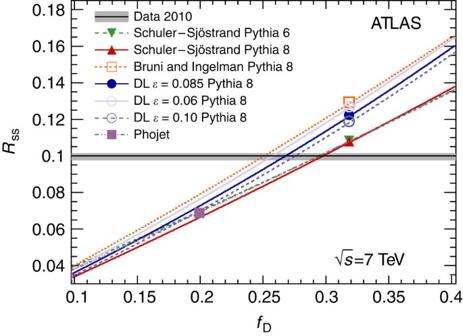Figure 1: Dependence of the fraction of single-sided events (Rss) on the relative diffractive contribution (fD). The ratio of the single-sided to inclusive event sampleRssas a function of the fractional contribution of diffractive events,fD, to the inelastic cross-section. The data value forRssis shown as the horizontal line with its systematic uncertainties (grey band). Also shown are predictions of several models as a function of an assumed value offD. For all three DL predictions, theα′ value is 0.25 GeV−2. The defaultfDvalues are indicated by the markers; they are 32.2% for all models except Phojet that uses 20.2%. Figure 1 compares the observed value of R ss to the predictions of several models as a function of f D . The intersection of the R ss value measured in data with the prediction is used as the central value of f D for each model. The systematic uncertainty on f D is determined by the maximum and minimum values consistent with the 1σ uncertainty on the data when varying the double- to single-dissociation event ratio between 0 and 1. The resulting value using the default DL model is Figure 1: Dependence of the fraction of single-sided events ( R ss ) on the relative diffractive contribution ( f D ). The ratio of the single-sided to inclusive event sample R ss as a function of the fractional contribution of diffractive events, f D , to the inelastic cross-section. The data value for R ss is shown as the horizontal line with its systematic uncertainties (grey band). Also shown are predictions of several models as a function of an assumed value of f D . For all three DL predictions, the α ′ value is 0.25 GeV −2 . The default f D values are indicated by the markers; they are 32.2% for all models except Phojet that uses 20.2%. Full size image Uncertainty on acceptance The acceptance calculation relies on the MC generators to provide an adequate description of the particle multiplicity in the acceptance region. 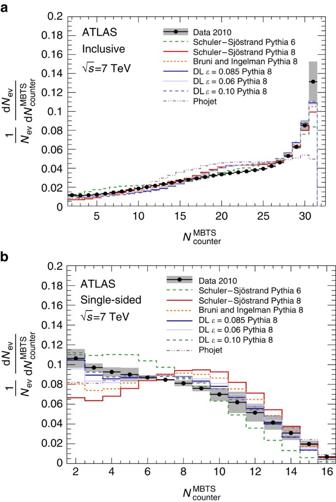Figure 2: MBTS multiplicity distributions. The MBTS multiplicity distribution in the data (filled circles) compared with MC expectations for the inclusive (a) and single-sided (b) samples for several MC models (histograms), using the fittedfDvalues. The band around the data indicates the systematic uncertainty due to the MBTS detector response and the amount of material in front of the MBTS detector. For all three DL predictions, theα′ value is 0.25 GeV−2. The validity of the MC description is assessed by examining the hit multiplicity in the MBTS detector in the inclusive and single-sided event samples as shown in Figure 2 . Whereas none of the generators gives a perfect description, the data lie between the models at low multiplicity that is most important for the measurement. Figure 2: MBTS multiplicity distributions. The MBTS multiplicity distribution in the data (filled circles) compared with MC expectations for the inclusive ( a ) and single-sided ( b ) samples for several MC models (histograms), using the fitted f D values. The band around the data indicates the systematic uncertainty due to the MBTS detector response and the amount of material in front of the MBTS detector. For all three DL predictions, the α ′ value is 0.25 GeV −2 . Full size image The inclusive sample, which is dominated by non-diffractive events, is reasonably well described by the MC. In addition, inclusive charged particle properties have been studied extensively in [37] , [38] that show that the Monte Carlo generators describe the data well. Differences in the acceptance for non-diffractive events were studied with several variations of the Pythia6 tuning parameters and were shown to be negligible. The single-sided sample is dominated by diffractive events. The default DL model describes it well, giving confidence in the diffractive modelling. We use the difference in the MC correction factor determined with Pythia8 and Pythia6 as the uncertainty due to the fragmentation model, leading to a 0.4% uncertainty on the cross-section. The maximum difference between the default DL model and all other models is taken as the uncertainty due to the underlying ξ distribution. Variations of α ′ have a negligible effect on the acceptance. Among all the models considered, the Phojet model gives the largest difference in the correction factor, leading to a 0.4% uncertainty on the cross-section. Inelastic cross-section The final result for the measured inelastic cross-section is calculated using the default DL model of ɛ =0.085 and α ′=0.25, which yields f D =26.9%, ɛ sel =98.77%, and Together with ɛ trig =99.98%, N =1,220,743, N BG =1,574 and this results in The systematic uncertainty includes all contributions discussed above and listed in Table 1 . The dominant uncertainty arises from the luminosity calibration and is quoted separately. Table 1 Systematic uncertainties. Full size table 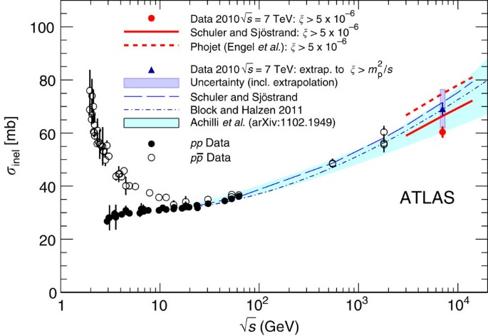Figure 3: The inelastic cross-section versus √s. The ATLAS measurement for ξ>5×10−6is shown as the red-filled circle and compared with the predictions of Schuler and Sjöstrand and Phojet for the same phase space. Data (filled circles forppdata and unfilled circles forpp̄data) from several experiments are compared with the predictions of theppinelastic cross-section from Schuler and Sjöstrand31(as used by Pythia), by Block and Halzen15and by Achilliet al.20An extrapolation from the measured range of ξ>5×10−6to the full inelastic cross-section using the acceptance of 87±10% is also shown (blue-filled triangle) based on the model by Donnachie and Landshoff forɛ=0.085 for dσ/dξ. The experimental uncertainty is indicated by the error bar whereas the total (including the extrapolation uncertainty) is represented by the blue-shaded area. The measurement is compared with the predictions in Figure 3 and Table 2 . The predictions by the Schuler-Sjöstrand model (66.4 mb) and the Phojet model (74.2 mb) are both higher than the data. The prediction of 51.8–56.2 mb by Ryskin et al . [17] and personal communication, is slightly lower than the data. Figure 3: The inelastic cross-section versus √ s . The ATLAS measurement for ξ>5×10 −6 is shown as the red-filled circle and compared with the predictions of Schuler and Sjöstrand and Phojet for the same phase space. Data (filled circles for pp data and unfilled circles for pp̄ data) from several experiments are compared with the predictions of the pp inelastic cross-section from Schuler and Sjöstrand [31] (as used by Pythia), by Block and Halzen [15] and by Achilli et al . [20] An extrapolation from the measured range of ξ>5×10 −6 to the full inelastic cross-section using the acceptance of 87±10% is also shown (blue-filled triangle) based on the model by Donnachie and Landshoff for ɛ =0.085 for d σ /d ξ . The experimental uncertainty is indicated by the error bar whereas the total (including the extrapolation uncertainty) is represented by the blue-shaded area. Full size image Table 2 Comparisons of the inelastic cross-section with predictions. Full size table To compare with previous measurements and analytic models, the fractional contribution to the inelastic cross-section of events passing the ξ>5×10 −6 cut is determined from the models and used to extrapolate the measurement to the full inelastic cross-section. This fraction is 87.3% for the default model of DL with ɛ =0.085 and α ′=0.25. The other models considered give fractions ranging from 96% (Phojet) to 86% (DL with ɛ =0.10). Recent calculations also yield values between 79 and 84% (ref. 17 ). Thus 87.3% is taken as the default value for this fraction and an uncertainty of 10% is taken because of the extrapolation uncertainty on the ξ -dependence. The resulting inelastic cross-section value is where the experimental uncertainty includes the statistical and experimental systematic errors, and the extrapolation uncertainty results from the uncertainty on the ξ -dependence of the cross-section. This result is shown in Figure 3 and compared with several theoretical predictions and a variety of data at lower √ s . The measurement within the kinematic range ξ>5×10 −6 is significantly lower than the predictions of Schuler and Sjöstrand and Phojet. The extrapolated value agrees within the large extrapolation uncertainty with the predictions from Pythia, which uses a power law dependence on √ s . It also agrees with Block and Halzen [15] (which has a logarithmic √ s dependence), and with other recent theoretical predictions that vary between 60 and 72 mb (refs 17 , 18 , 19 , 20 ). It should be stressed that this extrapolation relies on the prediction of the ξ -dependence of the cross-section. The measurement and a variety of theoretical predictions are also summarized in Table 2 . In conclusion, a first measurement of the inelastic cross-section has been presented for pp collisions at TeV with a precision of 3.5%. The measurement is limited to the kinematic range corresponding to the detector acceptance: ξ>5×10 −6 . Phenomenological predictions for both a power law dependence and a logarithmic rise of the cross-section with energy are consistent with the measurement. The ATLAS detector All measurements in this letter are made with the ATLAS detector, which is described in detail elsewhere [23] . Here the detector coordinate system and sub-detectors relevant to this measurement are described. ATLAS uses a right-handed coordinate system with its origin at the nominal interaction point in the centre of the detector and the z -axis aligned along the LHC beam pipe. The x -axis points from the interaction point to the centre of the LHC ring, and the y -axis points upward. Cylindrical coordinates ( r , φ ) are used in the transverse plane, φ being the azimuthal angle around the beam pipe. The pseudorapidity is defined in terms of the polar angle θ as η =−ln tan( θ /2). At the interaction point, the beam-line is surrounded by a tracking detector, which uses silicon pixel, silicon strip, and straw tube technologies, and is embedded in a 2-T magnetic field. The tracking system covers the pseudorapidity range | η |<2.5. It is surrounded by electromagnetic and hadronic calorimeters covering | η |<3.2, which are complemented by a forward hadronic calorimeter covering 3.1<| η |<4.9. MBTS detectors, the primary detectors used in this measurement, are mounted in front of the endcap calorimeters on both sides of the interaction point at z =±3.56 m and cover the range 2.09<| η |<3.84. Each side consists of 16 independent counters divided into two rings; the inner 8 counters cover the rapidity range 2.83<| η |<3.84 and the outer 8 counters cover the range 2.09<| η |<2.83. Each individual counter spans 45° of the azimuthal angle ( φ ), and 31 out of 32 counters were operational. The luminosity is measured using a Cherenkov light detector, LUCID, which is located at z =±17 m. The luminosity calibration has been determined during dedicated van der Meer beam scans to a precision of 3.4% using the technique described in ref. 36 . How to cite this article: The ATLAS Collaboration, Measurement of the inelastic proton–proton cross-section at TeV with the ATLAS detector. Nat. Commun. 2:463 doi: 10.1038/ncomms1472 (2011).